Microwave magnetoelectric effect via skyrmion resonance modes in a helimagnetic multiferroic Magnetic skyrmion, a topologically stable spin-swirling object, can host emergent electromagnetism, as exemplified by the topological Hall effect and electric-current-driven skyrmion motion. To achieve efficient manipulation of nano-sized functional spin textures, it is imperative to exploit the resonant motion of skyrmions, analogously to the role of the ferromagnetic resonance in spintronics. The magnetic resonance of skyrmions has recently been detected with oscillating magnetic fields at 1–2 GHz, launching a search for new skyrmion functionality operating at microwave frequencies. Here we show a microwave magnetoelectric effect in resonant skyrmion dynamics. Through microwave transmittance spectroscopy on the skyrmion-hosting multiferroic crystal Cu 2 OSeO 3 combined with theoretical simulations, we reveal nonreciprocal directional dichroism (NDD) at the resonant mode, that is, oppositely propagating microwaves exhibit different absorption. The microscopic mechanism of the present NDD is not associated with the conventional Faraday effect but with the skyrmion magnetoelectric resonance instead, suggesting a conceptually new microwave functionality. A magnetic skyrmion, a vortex-like spin-swirling object (see inset of Fig. 1a ), is now attracting considerable academic interests because it produces novel transport properties associated with its topological nature, such as topological Hall effect. Furthermore, as the size of magnetic skyrmions is typically 10–100 nm, they are potentially useful for next-generation spintronic devices with high information density [1] , [2] . Its crystalline form, the Skyrmion crystal (SkX), was studied theoretically [3] and was subsequently identified experimentally under a d.c. magnetic field H dc in B20-type metallic chiral-lattice magnets, such as MnSi, (Fe,Co)Si and FeGe, through the reciprocal-space and real-space observations [4] , [5] , [6] , [7] . In those systems, the coupling of conduction electrons to the skyrmions potentially allows their manipulation via electric currents [8] , [9] , [10] , [11] . Recently, SkX has been discovered also in the insulating chiral magnet Cu 2 OSeO 3 ( Fig. 1a ) [12] , [13] , [14] , [15] . This material hosts, as a multiferroic, a spin-texture mediated ferroelectric polarization P , pointing to a possibility for nominally joule-heating-free, electric-field control of skyrmions via the magnetoelectric (ME) coupling. In fact, a recent experiment has demonstrated that d.c. electric fields exert a torque on SkX and induce its tilting [16] . We extend the idea of eletromagnetic action of SkX in insulators into a dynamical regime and exploit a resonantly enhanced response of magnetism to electric fields (ME resonance) [17] , [18] . In this context, various resonant modes lying at microwave frequencies in the multiferroic Cu 2 OSeO 3 (ref. 19 ), such as the counterclockwise (CCW) and clockwise (CW) rotational modes ( Fig. 1b,c , respectively) and a breathing mode of skyrmion ( Fig. 1d ), would be promising candidates for the microwave ME resonance [19] , [20] , [21] , [22] . 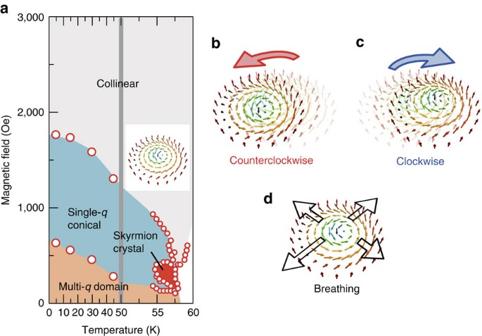Figure 1: Spin excitations via microwave in the multiferroics Cu2OSeO3. (a) Magnetic phase diagram underHdc||determined by magnetic a.c. susceptibility measurement. The vertical line represents a change in scale. Inset illustrates the spin texture of a skyrmion. Each arrow represents the net magnetic moment. (b–d) Schematic illustration of skyrmion resonant motions: (b) CCW and (c) CW modes, where the core of skyrmion rotates in such a sense, and (d) a breathing mode, where the skyrmion oscillatingly shrinks and enlarges. Figure 1: Spin excitations via microwave in the multiferroics Cu 2 OSeO 3 . ( a ) Magnetic phase diagram under H dc || determined by magnetic a.c. susceptibility measurement. The vertical line represents a change in scale. Inset illustrates the spin texture of a skyrmion. Each arrow represents the net magnetic moment. ( b – d ) Schematic illustration of skyrmion resonant motions: ( b ) CCW and ( c ) CW modes, where the core of skyrmion rotates in such a sense, and ( d ) a breathing mode, where the skyrmion oscillatingly shrinks and enlarges. Full size image In this work, we demonstrate the resonantly enhanced ME effect of these skyrmion modes through the microwave transmittance spectroscopy. This ME resonant character is accompanied by a new functionality that the absorption of an electromagnetic microwave by skyrmion motions depends on the direction of the incidence, that is, nonreciprocal directional dichroism (NDD). Furthermore, we address this phenomenon theoretically and find that the experimental results are well reproduced. The selection rule for the nonreciprocal effect is totally different from that of Faraday effect, indicating that the present NDD based on the skyrmion resonance may find novel application in microwave region. NDD via ME coupling The ME resonance in multiferroics involves the concomitant oscillations of P and magnetization M ; therefore, their interference with the E and H fields of electromagnetic wave may occur either constructively or destructively, which depends on the propagating vector k ω of electromagnetic wave [17] , [18] . When P and M oscillate constructively (destructively), the system can absorb electromagnetic waves more (less) efficiently. Thus, the ME resonance in multiferroics can lead to the nonreciprocal transmittance/absorption for a linearly polarized light: a phenomenon often called NDD. To detect microwave NDD as a hallmark of ME resonance, we carried out a two-port transmission spectroscopy on the coplanar waveguide circuit on which Cu 2 OSeO 3 was mounted ( Fig. 2a ; see also Methods). The microwave in the coplanar waveguide is basically a linearly polarized light and propagates as a TEM mode, that is, both the magnetic and electric field of the microwave are perpendicular to k ω . However, it should be noted that the polarization plane and hence the direction of H ω depend on the position in space: as shown in Fig. 2b , the H ω just above the center of signal line is parallel to the plane of the coplanar waveguide, whereas the H ω between the signal line and the ground is perpendicular to the plane. Thus, our experimental setup, which is based on the Voigt configuration ( H dc ┴ k ω ), includes not only H ω perpendicular to H dc but also H ω parallel to H dc ( Fig. 2b ). It follows that the present configuration using the coplanar waveguide allows all the resonant skyrmion motions; namely, two rotational modes (under H ω ┴ H dc ) and one breathing mode (under H ω || H dc ) [19] , [20] . 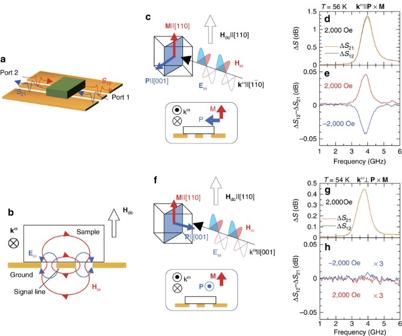Figure 2: Selection rule for NDD. (a) Schematic of the experimental setup. The sample size is roughly 1.5 × 3.5 × 0.5 mm3. The microwave propagates along the coplanar waveguide in both directions. (b) Electromagnetic-field distribution in the present setup using a coplanar waveguide, viewed from the direction of microwave propagation. (c,f) Schematic illustrations forkω||P×Mconfiguration (c) andkω┴P×Mconfiguration (f). The magnetic field is applied along [110], which leads toP||[001] andM||[110] (||Hdc) (ref.15). In the former configuration (c),kωis set to along [], whereas in the latter configuration (f),kωis set to along [001]. (d,g) Absorption spectra for microwave propagating from port 1 (2) to port 2 (1), ΔS21(ΔS12) for the cases ofkω||P×M(d) andkω┴P×M(g). (e,h) Nonreciprocal absorption spectra ΔS12−ΔS21under positive and negative magnetic fields for the cases ofkω||P×M(e) andkω┴P×M(h). Figure 2: Selection rule for NDD. ( a ) Schematic of the experimental setup. The sample size is roughly 1.5 × 3.5 × 0.5 mm 3 . The microwave propagates along the coplanar waveguide in both directions. ( b ) Electromagnetic-field distribution in the present setup using a coplanar waveguide, viewed from the direction of microwave propagation. ( c , f ) Schematic illustrations for k ω || P × M configuration ( c ) and k ω ┴ P × M configuration ( f ). The magnetic field is applied along [110], which leads to P ||[001] and M ||[110] (|| H dc ) (ref. 15 ). In the former configuration ( c ), k ω is set to along [ ], whereas in the latter configuration ( f ), k ω is set to along [001]. ( d , g ) Absorption spectra for microwave propagating from port 1 (2) to port 2 (1), Δ S 21 (Δ S 12 ) for the cases of k ω || P × M ( d ) and k ω ┴ P × M ( g ). ( e , h ) Nonreciprocal absorption spectra Δ S 12 −Δ S 21 under positive and negative magnetic fields for the cases of k ω || P × M ( e ) and k ω ┴ P × M ( h ). Full size image Experimental setup and selection rule To investigate the selection rule for NDD, we focus on the relation between k ω and P × M (refs 17 , 18 ). The important point is that the relation between k ω and P × M is relevant, whereas the direction of the H ω or E ω is irrelevant for the selection rule. From the symmetry point of view, the NDD is emergent unless P × M is orthogonal to k ω . However, there has been no report on the NDD associated with the ME resonance in a waveguide circuit, and we start with the verification of the selection rule in the field-induced collinear phase ( Fig. 1a ), where a ferrimagnetic resonance is expected via H ω ┴ H dc . To this end, we conducted the experiments under the two configurations: (i) k ω parallel to P × M ( Fig. 2c ) and (ii) k ω perpendicular to P × M ( Fig. 2f ). To achieve these configurations, H dc along [110] was chosen, where M and P appear along [110] and [001], respectively, leading to P × M || (ref. 15 ). Figure 2d,g presents the microwave absorption spectra measured under the ( k ω || P × M ( k ω || ) and k ω ┴ P × M ( k ω || ) configurations, respectively. The overall spectral shapes arising from the ferrimagnetic resonance are approximately similar to each other. Taking a closer look at Fig. 2d , however, one can find that the absorption of microwave propagating from port 2 to port 1 (denoted as Δ S 12 ) is slightly larger than the case of the opposite propagation, Δ S 21 . For clarity, the Δ S 12 −Δ S 21 spectrum under H dc =+2,000 Oe is plotted in Fig. 2e , where the nonreciprocal nature in the microwave absorption can be well discerned. To have a better understanding of the nonreciprocal absorption, we further investigated the Δ S 12 −Δ S 21 spectrum under H dc =−2,000 Oe, because reversing H dc (|| M ) should result in the sign reversal in P × M and hence in the Δ S 12 −Δ S 21 spectrum [17] , [18] . In fact, we obtained the sign-inverted Δ S 12 −Δ S 21 spectrum ( Fig. 2e ), in accord with the expectation. Contrastingly, the Δ S 12 −Δ S 21 spectrum under the configuration of k ω ┴ P × M turns out to exhibit no reciprocal nature with appreciable magnitude larger than the experimental accuracy ( Fig. 2g,h ), ~0.09%, whereas the NDD magnitude is ~3.3% in the k ω || P × M configuration (for the present definitions of the experimental accuracy and the NDD magnitude, see Methods). This observation is well accounted for by the expected selection rule for the NDD, namely, NDD disappears when k ω ┴ P × M , ensuring that the nonreciprocal microwave absorption observed here is traced back not to experimental artifacts but to NDD inherent in Cu 2 OSeO 3 . ME resonance of skyrmions The nonreciprocal microwave absorption is expected also in the SkX phase because there exists finite P × M . To see the microwave ME effect on the resonant skyrmion dynamics, we conducted the experiments with the k ω || P × M configuration and examined the magnetic-field dependence of the absorption spectra at 57 K. The results up to +1,000 Oe are displayed in Fig. 3a . In the collinear phase ( H dc >700 Oe) and conical phase ( H dc <250 Oe and 420 Oe< H dc <700 Oe), each absorption spectrum in the present frequency window comprises a single peak due to the resonant mode in each magnetic state; correspondingly, the NDD spectrum with a single peak is observed (for example, Fig. 3c ). In the intervening SkX phase at a intermediate field region, 250–420 Oe as determined by a.c. magnetic susceptibility ( Fig. 4a ), apparent two absorption bands are discerned around 1 GHz (open triangles in Fig. 3a ). The overall spectra in this region can be reproduced by a superposition of two Lorentzians multiplied by frequency, and a typical fitting result is displayed in Fig. 3d (for more details, see Methods). Among these two absorptions, the lower-lying mode can be unambiguously assigned to the CCW rotational mode of skyrmion [19] . At the resonance frequency of the lower-lying CCW mode, the NDD spectra are clearly observed ( Fig. 3e ), demonstrating an ME resonant character of CCW rotational motion of skyrmion. In contrast, the origin of the higher-lying absorption in the SkX phase ( Fig. 3d ) has remained elusive, partly because the resonance frequency is quite close to that in the possible remnant domains of the conical phase. Furthermore, the CW rotational mode ( Fig. 1c ; allowed when H ω ┴ H dc ) and the breathing mode ( Fig. 1d ; allowed when H ω || H dc ) of skyrmion is anticipated to take place and be overlapped in this region, because the two modes have similar resonance frequencies [19] , [20] and our experimental setup produces a superposition of two linearly polarized lights, that is, H ω ┴ H dc and H ω || H dc , as illustrated in Fig. 2b . Focusing on the NDD spectra under a positive magnetic field, however, we found that the higher-lying absorption in the SkX phase exhibits the negative NDD spectra ( Fig. 3e ), whereas only the positive NDD spectra are observed in other magnetic phases ( Fig. 3c ). This clearly indicates that the higher-lying absorption cannot share the same origin with that observed in the conical phase but should be attributed to the resonant skyrmion dynamics distinct from the CCW rotational motion. 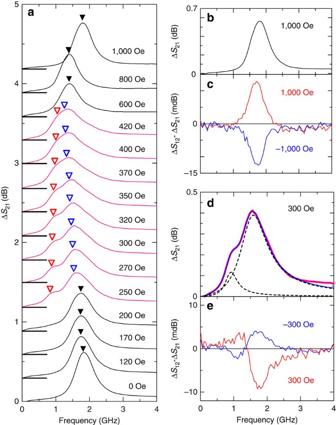Figure 3: ME resonance spectra and NDD. (a) Magnetic-field dependence of the absorption spectra at 57 K for thekω||P×Mconfiguration (that is,P||[001],M||Hdc||[110] andkω||[]). Each spectrum is shifted upward for clarity; the offset levels are indicated by horizontal solid lines. The spectra in the SkX phase are highlighted by red colour. The triangles indicate the resonant frequencies. (b,d) Microwave absorption spectra atHdc=1,000 and 300 Oe, which corresponds to collinear and SkX, respectively. In (d), the results of two-peak fitting are also shown in addition to the raw data (red line): the broken lines represent each component, and the blue solid line is a sum of them. (c,e) Nonreciprocal absorption spectra atHdc=±1,000 Oe and ±300 Oe. Figure 3: ME resonance spectra and NDD. ( a ) Magnetic-field dependence of the absorption spectra at 57 K for the k ω || P × M configuration (that is, P ||[001], M || H dc ||[110] and k ω ||[ ]). Each spectrum is shifted upward for clarity; the offset levels are indicated by horizontal solid lines. The spectra in the SkX phase are highlighted by red colour. The triangles indicate the resonant frequencies. ( b , d ) Microwave absorption spectra at H dc =1,000 and 300 Oe, which corresponds to collinear and SkX, respectively. In ( d ), the results of two-peak fitting are also shown in addition to the raw data (red line): the broken lines represent each component, and the blue solid line is a sum of them. ( c , e ) Nonreciprocal absorption spectra at H dc =±1,000 Oe and ±300 Oe. 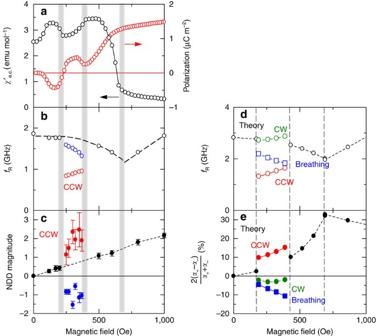Figure 4: Comparison between experiment and theory of the skyrmion ME resonance. (a–c) Magnetic-field dependence of a.c. magnetic susceptibility forHdc||[110] (a), the resonance frequencyωR(b) and the normalized magnitude of nonreciprocal absorption for thekω||P×Mconfiguration (that is,P||[001],M||Hdc||[110] andkω||[]). (c) Ina, the electric polarization profile is also presented. Broken line inbis a guide to the eyes. (d,e) Theoretical simulation of the magnetic-field dependence of the resonance frequenciesωR(d) and the magnitudes of the NDD normalized by the absorption coefficient (e). The thick vertical lines ina–cand the broken vertical lines indanderepresent the boundaries between different magnetic phases: from low to high fields, the magnetic phases are helical, SkX, conical and collinear. The error bars inFig. 4care associated with the variance of the nonreciprocal absorption in the off-resonant frequency range. For more details, see Methods. To check the reproducibility, the experiments were conducted four times, and the results were found to be reproducible. Full size image Figure 4: Comparison between experiment and theory of the skyrmion ME resonance. ( a – c ) Magnetic-field dependence of a.c. magnetic susceptibility for H dc ||[110] ( a ), the resonance frequency ω R ( b ) and the normalized magnitude of nonreciprocal absorption for the k ω || P × M configuration (that is, P ||[001], M || H dc ||[110] and k ω ||[ ]). ( c ) In a , the electric polarization profile is also presented. Broken line in b is a guide to the eyes. ( d , e ) Theoretical simulation of the magnetic-field dependence of the resonance frequencies ω R ( d ) and the magnitudes of the NDD normalized by the absorption coefficient ( e ). The thick vertical lines in a – c and the broken vertical lines in d and e represent the boundaries between different magnetic phases: from low to high fields, the magnetic phases are helical, SkX, conical and collinear. The error bars in Fig. 4c are associated with the variance of the nonreciprocal absorption in the off-resonant frequency range. For more details, see Methods. To check the reproducibility, the experiments were conducted four times, and the results were found to be reproducible. Full size image Comparison with the numerical calculation To identify the higher-lying resonant skyrmion dynamics with the ME character, we carried out a numerical calculation at zero temperature and examined the magnetic-field dependence of the resonance frequency, ω R ( H dc ), and the magnitude of NDD. Here we employed a model Hamiltonian that is used in Mochizuki and Seki [22] (for details, see Methods) and known to reproduce the SkX under a magnetic field. The experimental results are plotted in Fig. 4b,c , whereas the numerical results are in Fig. 4d,e . Concerning the resonant modes in the helical, conical and collinear phases and the lower-lying CCW rotational mode in the SkX phase, we found that ω R ( H dc ) exhibits a good agreement between the experiment and theory; moreover, the magnetic-field evolutions of NDD are also consistent at least on a qualitative level ( Fig. 4c,e ). Regarding the higher-lying mode, the experimental ω R ( H dc ) ( Fig. 4b ) coincides with that of the breathing mode in the simulations rather than the CW rotational mode ( Fig. 4d ); therefore, the skyrmion motion at the higher-lying absorption is ascribed to the breathing mode. It is worth mentioning that not only the behaviour of ω R ( H dc ) but also the signs of NDD are consistent between the experiments and theory in all the magnetic phases. A large difference in magnitude of NDD between the experiments ( Fig. 4c ) and the zero-temperature simulations ( Fig. 4e ) can be reasonably attributed to a thermal contraction of magnetic moments at a measurement temperature (~57 K) close to the paramagnetic phase boundary. As a whole, the magnitude of NDD increases with a magnetic field ( Fig. 4c ); this may be explained qualitatively by increase in the net magnetization M and electric polarization P . However, some observations should be interpreted beyond the phenomenological understanding of NDD based on P × M . First, the NDD does not change its sign when P is reversed. The sign of P is negative in the lower-field conical phase ( H dc <250 Oe) and positive in the higher-field conical phase (420 Oe< H dc <700 Oe), whereas the NDD is positive for the both phases ( Fig. 4c ). Second, although the magnitudes of P and M in the SkX phase is not so different from those in the conical phases, the NDD signal in the SkX phase shows an appreciable enhancement. Finally, the sign and magnitude in NDD are different between the different resonant skyrmion motions, for example, CCW rotational mode versus breathing mode. These observations clearly suggest that understanding of the entanglement between local electric and magnetic dipoles and their dynamics is crucial for the emergent microwave NDD. In conclusion, we have conducted the microwave transmittance spectroscopy and numerical simulation on the multiferroic helimagnet Cu 2 OSeO 3 to prove the ME character of the skyrmion resonant mode by observing microwave NDD. It has been confirmed that the selection rule, k ω || P × M , holds for the microwave NDD effect as well; the NDD vanishes when k ω ┴ P × M . The theoretical simulations have successfully reproduced the experimental observations regarding the sign and the magnetic-field dependence of NDD. This skyrmion ME effect will open a new avenue for the skyrmion-based microwave functionalities. Sample preparation and characterization Single crystal of Cu 2 OSeO 3 was prepared by chemical vapour transport [12] . Magnetic a.c. susceptibility was measured with a SQUID magnetometer (MPMS; Quantum Design). Microwave transmittance spectroscopy The broadband microwave transmission spectroscopy was carried out by using a vector network analyser (E8363C; Agilent Technology), with the sample mounting on a coplanar waveguide. The H dc (|| M ) was applied along [110] throughout the experiments, in which configuration the finite P appears along [001], orthogonal to H dc (ref. 15 ). We define the absorption spectrum due to magnetic excitation Δ S 21(12) ( ω , H dc ) as Δ S 21(12) ( ω , H dc )= S 21(12) ( ω , 5,000 Oe)− S 21(12) ( ω , H dc ), where S 21(12) ( ω , H dc ) denotes a transmittance spectrum at H dc : the resonance frequency at 5,000 Oe is beyond 8 GHz and can therefore be regarded as the system background as far as our frequency window (0.01–6 GHz) is considered. To avoid the possible effect of hysteresis, we first applied H dc up to 5,000 Oe and then decreased H dc to the target field. The definition of the resonance frequency ω R and the NDD magnitude are as follows: at a given magnetic field in the conical or ferrimagnetic phases (for example, Fig. 3b ), we define ω R as the peak frequency in the absorption spectra and the magnitude of NDD as . In the SkX phase (for example, Fig. 3d ), we found that the overall absorption spectra can be well reproduced by a superposition of two Lorentzians multiplied by frequency, that is, , where A , B , C , D , ω R1 and ω R2 are all fitting parameters, as shown in Fig. 3d . The errors in estimating each NDD magnitude were defined as the variance of Δ S 12 −Δ S 21 in the off-resonant regime divided by the peak value of each component. Numerical calculation of the dynamical ME tensor We employed a two-dimensional classical Heisenberg model that contains the ferromagnetic-exchange interaction, the Dzyaloshinskii–Moriya interacion and the Zeeman coupling to H dc . The parameters in the Hamiltonian were chosen so as to reproduce experimental values of the helical period and the critical magnetic fields that separate the different magnetic phases [12] . A local polarization at each site was evaluated within the d–p hybridization model [15] , [23] , [24] , and we calculated the temporal evolution of spins and polarizations after applying a microwave pulse by solving the Landau–Lifshitz–Gilbert equation numerically. Then, we obtained their Fourier tranforms and derived the ME tensors. For more details, see Mochizuki and Seki [22] . How to cite this article: Okamura, Y. et al . Microwave magnetoelectric effect via skyrmion resonance modes in a helimagnetic multiferroic. Nat. Commun. 4:2391 doi: 10.1038/ncomms3391 (2013).